Broadband omnidirectional antireflection coating based on subwavelength surface Mie resonators Reflection is a natural phenomenon that occurs when light passes the interface between materials with different refractive index. In many applications, such as solar cells or photodetectors, reflection is an unwanted loss process. Many ways to reduce reflection from a substrate have been investigated so far, including dielectric interference coatings, surface texturing, adiabatic index matching and scattering from plasmonic nanoparticles. Here we present an entirely new concept that suppresses the reflection of light from a silicon surface over a broad spectral range. A two-dimensional periodic array of subwavelength silicon nanocylinders designed to possess strongly substrate-coupled Mie resonances yields almost zero total reflectance over the entire spectral range from the ultraviolet to the near-infrared. This new antireflection concept relies on the strong forward scattering that occurs when a scattering structure is placed in close proximity to a high-index substrate with a high optical density of states. Many different ideas have been developed over the years to reduce reflection in optical and optoelectronic devices [1] , [2] . A single transparent dielectric layer is commonly used as an antireflection (AR) coating. On the basis of destructive interference between the incident and reflected light, perfect optical impedance matching can be achieved for one specific wavelength [3] . Micron-sized pyramidal surface texturing is also widely used in, for example, crystalline silicon solar cells [4] , [5] . The angular randomization of the scattered light at the surface can increase light absorption in an optical medium up to a factor of 4 n 2 , where n is the refractive index of the medium. [6] , [7] Surface structures composed of periodic or random arrays of semiconductor nanowires and nanopyramids have also proven to reduce reflection over a broad range of wavelengths and angles of incidence [7] , [8] , [9] , [10] , [11] , [12] , [13] , [14] , [15] . The reduced reflection is caused by multiple scattering of light as well as adiabatic coupling due to a gradually increasing refractive index towards the substrate surface [16] , [17] , [18] , [19] , [20] , [21] . Recently, we have shown that optimized arrays of metal nanoparticles reduce reflection of silicon in the range of wavelengths relevant for solar applications [22] , [23] . Preferential forward scattering by the plasmonic point scatterers [24] strongly reduces the reflection, thus allowing almost perfect impedance matching of sunlight into a Si wafer. Here we present an entirely new concept to eliminate reflection from a silicon wafer that makes use of much simpler nanostructures than the ones reported before, does not involve metals, and can be applied to any high-index material. It is based on the fact that dielectric nanoscatterers possess geometrical Mie resonances with scattering cross-sections larger than the geometrical ones [25] , [26] . A recent paper by Cao et al . [27] has shown that Mie resonances provide a very efficient mechanism for light absorption in Si nanowire-based solar cells. In that work, however, Si nanowires were on a glass substrate and only absorption in the nanowires was considered. In this paper, we demonstrate that light that is stored in Mie resonances can also be very efficiently coupled to a Si substrate. From a fundamental point of view this light coupling mechanism, based on weak (lossy) Mie resonances, is entirely different than all other methods commonly known in the field of AR coatings. We demonstrate experimentally that an array of low aspect-ratio Si nanocylinders etched into a Si wafer shows an average reflectivity as low as 1.3% in the 450–900 nm spectral range. The strongly reduced reflectivity is observed for angles of incidence up to 60°. The monolithic nature of the nanostructures makes this novel AR concept easily applicable to a wide range of devices, including (ultra-thin) solar cells based on any high-index semiconductor [28] . Author contributions P.S. did the theoretical modelling and the reflectivity measurements. M.A.V. coordinated the fabrication of samples at Philips Research. A.P. supervised the research. All authors contributed to the editing of the manuscript. 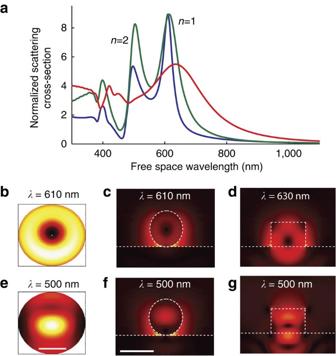Figure 1: Mie scattering on a Si wafer. (a) Scattering cross-sections, normalized to the geometrical cross-section, for a Si sphere in air (blue), a Si sphere on a Si substrate (green) and a Si cylinder on a Si substrate (red). The spheres have diameterd=150 nm, the cylinder has an in-plane diameter of 150 nm and height of 100 nm. Mie resonances of first (n=1) and second (n=2) order are indicated in the figure. (b–g) Electric field intensity (colour scale) in a cross-section of the particle for a sphere in air (b,e), a sphere on substrate (c,f) and a cylinder on substrate (d,g), for Mie modes of first (b–d) and second (e–g) order. The wavelengths considered for these calculations are indicated in each panel. The field distribution for the cylinder at resonance overlaps with the substrate, thus introducing a loss channel for the light confined in the particle that broadens the resonances. Plots for a sphere in air are calculated with Mie theory; plots for particles on a substrate are simulated. The scale bar inerepresents 50 nm, and refers tobande. The scale bar infrepresents 150 nm and refers toc,d,fandg. Mie scattering on a Si substrate Figure 1a shows the calculated scattering cross-section spectra, normalized to the geometrical cross-section, for a Si sphere in air (blue) and a Si sphere (green) and cylinder (red) on top of a Si substrate. The scattering spectrum for the sphere in air shows two distinct resonances corresponding to the first- and second-order Mie modes. These geometrical resonances reflect the fact that the particle acts as a nano-cavity for light. The scattering cross-section at resonance is more than eight times larger than the geometrical cross-section, and the cavity quality factor ( Q =10) is determined by radiation losses from the cavity mode. The two scattering resonances are clearly visible when a Si substrate is introduced below the spherical particle (green line), indicating only weak coupling of the well-confined Mie modes to the substrate. However, when a cylindrical nanoparticle is placed on the Si substrate, the resonances broaden and merge into a broadband feature (red line). This behaviour is due to the introduction of a leaky channel into the substrate for the light that is resonantly confined in the particle. To understand this mechanism, Figure 1b–g show the calculated distribution of light (electric field intensity, colour scale) inside a Si sphere in air ( Fig. 1b,e ), a Si sphere on a Si substrate ( Fig. 1c,f ) and a Si cylinder on a Si substrate ( Fig. 1d,g ) for Mie modes of first ( Fig. 1b–d ) and second ( Fig. 1e–g ) order. Comparison of the field distributions shows that the geometrical modes inside a spherical Si particle are nearly unaffected by the presence of the substrate and light in both cases is well confined inside the particle. However, for a cylindrical particle the field distribution of the Mie resonances has a clear overlap with the Si substrate. Both direct near-field absorption in the substrate and radiative emission into the substrate introduce a loss channel for the light confined in the particle, thus yielding broadening of the resonances in the scattering cross-section spectrum ( Q ~5; Supplementary Fig. S1 ). Figure 1: Mie scattering on a Si wafer. ( a ) Scattering cross-sections, normalized to the geometrical cross-section, for a Si sphere in air (blue), a Si sphere on a Si substrate (green) and a Si cylinder on a Si substrate (red). The spheres have diameter d =150 nm, the cylinder has an in-plane diameter of 150 nm and height of 100 nm. Mie resonances of first ( n =1) and second ( n =2) order are indicated in the figure. ( b – g ) Electric field intensity (colour scale) in a cross-section of the particle for a sphere in air ( b , e ), a sphere on substrate ( c , f ) and a cylinder on substrate ( d , g ), for Mie modes of first ( b – d ) and second ( e – g ) order. The wavelengths considered for these calculations are indicated in each panel. The field distribution for the cylinder at resonance overlaps with the substrate, thus introducing a loss channel for the light confined in the particle that broadens the resonances. Plots for a sphere in air are calculated with Mie theory; plots for particles on a substrate are simulated. The scale bar in e represents 50 nm, and refers to b and e . The scale bar in f represents 150 nm and refers to c , d , f and g . Full size image Ultra-low reflectivity The field distributions in Figure 1b–g suggest that a cylindrical Si nanoparticle can effectively couple light into a Si substrate. To study this further we perform simulations of the reflectance spectra of cylindrical nanopillar (NP) arrays with different NP dimensions. 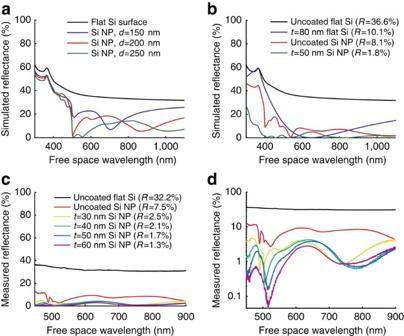Figure 2: Ultra-low reflectivities. (a) Simulated reflection spectra from a regular square array of Si NPs spaced by 500 nm, for cylinder diameters of 150 (blue), 200 (red) and 250 nm (green) with a height of 150 nm. Reflectance from a flat Si surface is also shown for comparison (black). The Si NP arrays reduce the reflectivity over the entire spectrum. The broad dip in reflectivity that redshifts for increasing particle diameter is due to enhanced forward scattering from the Mie resonances in the particle. (b) Simulated reflection spectra for a bare flat Si substrate (black), a flat Si substrate coated with a standard Si3N4antireflection coating (blue, thicknesst=80 nm), a Si surface with bare Si nanostructures on top (red) and a Si surface with Si nanostructures on top coated with an optimized Si3N4layer (green,t=50 nm). For each configuration the average reflectivity,R, weighted with the AM1.5 solar spectrum in the 300–1,100 nm spectral range, is indicated. (c) Measured total reflectivity of a bare Si wafer (black), an uncoated Si NP array (red) and four Si NP array coated with Si3N4layers of different thicknesses,t(colours). The Si NPs have a diameter of 125 nm, height of 150 nm and are spaced by 450 nm. For each configuration the average reflectivity,R, weighted with the AM1.5 solar spectrum in the 450–900 nm spectral range, is indicated. Reflectance is reduced over the entire spectral range, due to coupling of the Mie resonant scattering to the Si substrate. (d) The same reflectivity data plotted in logarithmic scale. Individual curves are described in legend toFigure 3c. The effect of the Mie resonance is visible in the broad dip in reflectivity observed in the 700–800 nm range. Figure 2a shows the simulated total reflectance spectra from a square array of Si NPs spaced by 500 nm, for cylinder diameters of 75, 100 and 125 nm. The reflectance from a bare flat Si surface (35–60%) is also shown for comparison (black line). The data in Figure 2a show that the dielectric particle array reduces the reflectance of a Si surface over the entire spectral range shown. The key role of the Mie resonances in the reduced reflection is clear from the fact that broad reflection dips are observed on resonance, at wavelengths (700, 830 and 1,000 nm) that increase with NP diameter (150, 200 and 250 nm). This redshift for increasing diameter is similar to that observed for Mie resonances for isolated particles with increasing diameter ( Supplementary Fig. S1 ). The sharp decrease in reflectivity at the wavelength of 500 nm, that is, equal to the array pitch, is explained by a Rayleigh anomaly [29] from the grating formed by the regular array of nanoparticles ( Supplementary Fig. S2 ). Figure 2: Ultra-low reflectivities. ( a ) Simulated reflection spectra from a regular square array of Si NPs spaced by 500 nm, for cylinder diameters of 150 (blue), 200 (red) and 250 nm (green) with a height of 150 nm. Reflectance from a flat Si surface is also shown for comparison (black). The Si NP arrays reduce the reflectivity over the entire spectrum. The broad dip in reflectivity that redshifts for increasing particle diameter is due to enhanced forward scattering from the Mie resonances in the particle. ( b ) Simulated reflection spectra for a bare flat Si substrate (black), a flat Si substrate coated with a standard Si 3 N 4 antireflection coating (blue, thickness t =80 nm), a Si surface with bare Si nanostructures on top (red) and a Si surface with Si nanostructures on top coated with an optimized Si 3 N 4 layer (green, t =50 nm). For each configuration the average reflectivity, R , weighted with the AM1.5 solar spectrum in the 300–1,100 nm spectral range, is indicated. ( c ) Measured total reflectivity of a bare Si wafer (black), an uncoated Si NP array (red) and four Si NP array coated with Si 3 N 4 layers of different thicknesses, t (colours). The Si NPs have a diameter of 125 nm, height of 150 nm and are spaced by 450 nm. For each configuration the average reflectivity, R , weighted with the AM1.5 solar spectrum in the 450–900 nm spectral range, is indicated. Reflectance is reduced over the entire spectral range, due to coupling of the Mie resonant scattering to the Si substrate. ( d ) The same reflectivity data plotted in logarithmic scale. 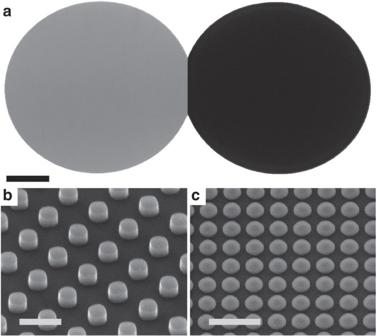Figure 3: Black silicon. (a) Photograph of a bare flat 4-inch Si wafer (left) and a 4-inch Si wafer fully imprinted with an optimized (250 nm diameter, 150 nm height, 450 nm pitch) Si NP array and overcoated with a 60-nm-thick Si3N4layer (right). Scale bar represents 1 inch. (b) Scanning electron microscopy image taken under an angle of 40° of a bare Si NP array (scale bar represents 500 nm) and (c) a Si NP array coated with a 60-nm-thick Si3N4layer (scale bar represents 1 μm). Individual curves are described in legend to Figure 3c . The effect of the Mie resonance is visible in the broad dip in reflectivity observed in the 700–800 nm range. Full size image The strong coupling of light on resonance is explained by the strong forward scattering of light from the resonant Mie scatterers, due to the high optical mode density of the high-index Si substrate [30] . The resonant nature of this effect leads to a large cross-section, so that even an array of scatterers covering only 30% of the surface area leads to nearly complete interaction with the incoming plane wave. Figure 2b shows the simulated reflectivity spectra for a bare flat Si substrate (black), a flat Si substrate coated with a standard 80 nm Si 3 N 4 antireflection coating (blue), a Si surface with bare Si NP on top (red) and a Si surface with Si NP on top coated with a 50 nm Si 3 N 4 layer (green). Given its index ( n =2.0), Si 3 N 4 is the optimum AR coating for a Si wafer ( n =3.5–4.0 in the visible-to-near-infrared spectral range). As can be seen in the figure, it only leads to vanishing reflectivity for a specific wavelength (650 nm in Fig. 2b ), determined by the Si 3 N 4 layer thickness. The bare array of Si NPs shows a broadband reduced reflectivity spectrum that is lower than that for the standard AR coating above 850 nm and below 550 nm, and higher in the range 550–850 nm. Both spectra show a large increase in reflectivity for wavelengths below 500 nm. A Si 3 N 4 layer with properly chosen thickness can be used as a coating, conformal to the nanostructures, to compensate for the losses in this spectral region. The reflectance spectrum from a coated array of NPs ( Fig. 2b , green) shows that reflectivity can be reduced down to <2% over the entire spectral range from 400 to 1,100 nm, with the exception of a small peak around 650 nm. The low reflectivity stems from the combined effect of the strongly coupled Mie resonances in the red and near-infrared part of the spectrum and the interference antireflection effect from the Si 3 N 4 layer, tuned for the blue part of the spectrum. Figure 2b also shows the average reflectivities for each configuration, obtained by weighting over the AM1.5 solar spectrum in the 300–1,100 nm spectral range. As can be seen, both coated (1.8%) and uncoated NP arrays (8.1%) show lower reflectivity than the standard 80 nm Si 3 N 4 coating (10.3%). Black silicon The AR properties of Si NP arrays have been studied experimentally using Si(100) wafers, on which square arrays of Si nanocylinders (250 nm diameter, 150 nm height, 450 nm pitch) were fabricated using substrate conformal soft-imprint lithography in combination with reactive ion etching (RIE). The total hemispherical reflectivity was measured using an integrating sphere, with an angle of incidence (AOI) of 8° off the surface normal. Figure 2c shows the measured total reflectivity spectrum of a bare Si wafer (black), of a bare Si NP array (red) and four Si NP arrays coated with different Si 3 N 4 layer thicknesses (green to purple colour lines). All geometries show a reduced reflectivity with respect to the bare Si wafer, over the entire spectral range. The array coated with a 60-nm thick Si 3 N 4 layer (purple line) shows a reflectivity <3% over the entire spectral range 450–900 nm. The AM1.5-averaged reflectance from a bare Si substrate (32.2%, black) is reduced to 7.5% by pattering the Si surface with an optimized Si NP array (red). Combining Si NPs and a Si 3 N 4 coating leads to an average reflectivity as low as 1.3% (purple). This value is in excellent agreement with the calculated data in Figure 2b , taking into account the different spectral range over which the average reflectivity is calculated ( Supplementary Figs S3 and S4 ). Figure 2d shows the same reflectivity spectra plotted on a logarithmic scale. The broad dip in the reflectivity spectra at wavelengths between 650 and 850 nm is attributed to the first-order coupled Mie resonances. The sharp dips at a wavelength of about 510 nm are consistent with a Rayleigh anomaly for light incident with an AOI of 8° ( Supplementary Fig. S5 ). With the reflection of light effectively vanished, light is then either transmitted into the Si substrate or absorbed in the NPs. For example, for silicon in the 800–1,000 nm spectral range the linear absorption over the thickness of the nanocylinders is <1%; it is enhanced in the cavity by the quality factor Q~3. Indeed, simulations ( Supplementary Fig. S6 ) show that in this spectral range absorption in the NPs is negligible and the NPs behave as almost pure scatterers (that is, the albedo is almost 1). For the ultraviolet/blue spectral range, Si is strongly absorbing and light is absorbed inside the Si nanocylinders. Indeed, an optimized solar cell design based on substrate-coupled Mie resonators will have the p–n junction integrated inside the nanoparticles, which can easily be done using gas-phase doping. Figure 3a shows a photograph of a bare flat 4-inch Si wafer compared to a 4-inch Si wafer that has been patterned over the entire wafer area with an optimized Si NP array and overcoated with a 60-nm-thick Si 3 N 4 layer. The photograph shows a clear visual effect of the reduced reflectivity due to the patterning of the Si wafer surface with resonant Mie scatterers. Figure 3 shows a scanning electron microscopy image of a bare ( Fig. 3b ) and a 60-nm Si 3 N 4 -coated ( Fig. 3c ) NP array. The sample shown in Figure 3 was fabricated using interference lithography and soft-imprint lithography, demonstrating that this new AR coating design can be applied at large-area using standard inexpensive processes. Figure 3: Black silicon. ( a ) Photograph of a bare flat 4-inch Si wafer (left) and a 4-inch Si wafer fully imprinted with an optimized (250 nm diameter, 150 nm height, 450 nm pitch) Si NP array and overcoated with a 60-nm-thick Si 3 N 4 layer (right). Scale bar represents 1 inch. ( b ) Scanning electron microscopy image taken under an angle of 40° of a bare Si NP array (scale bar represents 500 nm) and ( c ) a Si NP array coated with a 60-nm-thick Si 3 N 4 layer (scale bar represents 1 μm). Full size image Angle-resolved reflectivity To be relevant for, for example, photovoltaic applications, an AR coating must show low reflectivity over a wide range of angles of incidence and for both polarizations of light. 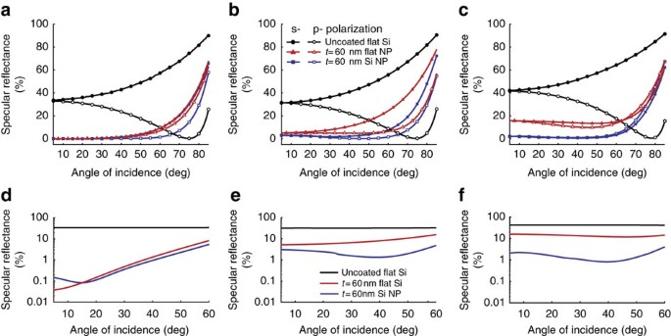Figure 4: Angle resolved reflectivity. Specular reflectivity measured as a function of AOI, for wavelengths of 514 nm (a,d), 632 nm (b,e) and 405 nm (c,f). Panels in the top row show results for s- (solid symbols) and p-polarized (open symbols) incident beam, whereas the bottom row show an average of s- and p-polarizations, plotted on a logarithmic scale. In each graph, reflectivities from a bare Si wafer (black lines), a 60-nm standard Si3N4coating (red) and a coated NP array (blue) are shown. The excellent AR properties of Si NP arrays are maintained over the entire range of AOI from −60° to +60°. Figure 4 shows the specular reflectivity measured as a function of AOI, for wavelengths of 514 nm ( Fig. 4a,d ), 632 nm ( Fig. 4b,e ) and 405 nm ( Fig. 4c,f ). Figure 4a–c shows reflectance for s- (solid symbols) and p-polarized (open symbols) incident beams, whereas Figure 4d–f shows the average reflectivity for s- and p-polarizations, plotted on a logarithmic scale. In each graph, reflectivities from a bare Si wafer (black lines), a flat Si wafer with a 60-nm standard Si 3 N 4 coating (red) and a 60-nm-thick Si 3 N 4 -coated NP array (blue) are shown. At a wavelength of 514 nm, the 60 nm standard coating and the coated NP array show a total reflectivity for near-normal incidence of 0.1 and 0.05%, respectively ( Supplementary Fig. S3a ). Figure 4a shows that for both samples and polarizations the reflectivity remains below 1% in a wide range of AOI. While no difference between the standard coating and the Si NP array is seen for the s-polarization, the Si NP array shows lower reflection of p-polarized light at large angles. Averaging the two polarizations ( Fig. 4d ) yields similar results for the standard and the Si NP coatings, with better AR properties from the latter for angles above 14 ° . At wavelengths of 632 nm ( Fig. 4b ) and 405 nm ( Fig. 4c ), the Si NP array shows lower reflectivity than the standard Si 3 N 4 coating, for both polarizations and over the entire range of AOI. As Figure 4e and f shows, the low reflectivity from the coated Si NP array is maintained over the entire angular range up to 60°. Figure 4: Angle resolved reflectivity. Specular reflectivity measured as a function of AOI, for wavelengths of 514 nm ( a , d ), 632 nm ( b , e ) and 405 nm ( c , f ). Panels in the top row show results for s- (solid symbols) and p-polarized (open symbols) incident beam, whereas the bottom row show an average of s- and p-polarizations, plotted on a logarithmic scale. In each graph, reflectivities from a bare Si wafer (black lines), a 60-nm standard Si 3 N 4 coating (red) and a coated NP array (blue) are shown. The excellent AR properties of Si NP arrays are maintained over the entire range of AOI from −60° to +60°. Full size image Subwavelength resonant Mie scatterers at the surface of a Si wafer cause the reflection of light from the wafer to vanish. The resonant Mie modes have large scattering cross-sections, leading to strong interaction with the incident light. Coupling of these modes to the substrate leads to strong preferential forward scattering due to the high-mode density in the high-index substrate. Full-wafer Si nanocylinder arrays were fabricated using a soft-imprint technique capable of large scale, high-fidelity surface patterning. Total reflectance spectroscopy shows an average reflectivity of only 1.3% over the 450–900 nm spectral range. The strongly reduced reflectivity is observed for a broad range of angles of incidence up to ±60°. Owing to the monolithic nature of the Mie scatterers, this novel antireflection concept is easily applicable to any high-index material. It can readily find application in solar cells, including thin-film designs on which the standard texturing cannot be applied. Numerical calculations The scattering cross-section spectra and field distributions shown in Figure 1 have been calculated using Mie theory [26] (blue line in Fig. 1a and Fig. 1b and e ) and finite-difference time-domain (FDTD) calculations (green and red lines in Fig. 1a , and Fig. 1c,d,f and g ). For a definition of scattering cross-section please refer to ref. 26 , chapter 2. A commercial software package was used to perform FDTD calculations [31] . A simulation box size of 1×1×0.8 ìμm with perfectly matched layer conditions on every boundary was used. The light source was a broadband (300–1100 nm) plane wave, with normal incidence to the substrate. The mesh grid was set to 5 nm over the entire simulation volume, with a refinement (1 nm) over the volume occupied by the particle. A total-field scattered-field method was used to directly calculate the scattered power by means of frequency-domain transmission monitors positioned in the scattered field region. A two-dimensional frequency-domain field monitor cross-cutting the particle in its centre was used to calculate the electric field intensity distribution (as shown in Fig. 1c, d, f and g ). FDTD simulations were also used to study the AR properties of Si NP arrays on a Si substrate ( Fig. 2a and b). In this case, the box size was equal to p × p ×0.6 μm, where p is the array pitch, and periodic boundary conditions were used in the in-plane directions. The reflectivity spectra were directly calculated with a frequency-domain transmission monitor placed above the plane-wave source. Optical constants of Si and Si 3 N 4 were taken from the literature [32] . Fabrication of Si NP arrays Substrate conformal imprint lithography was used to fabricate large area Si NP arrays. This soft-imprint fabrication technique is capable of large-scale, high-fidelity surface patterning and is fully compatible with standard techniques used in, for example, solar cell manufacturing. It uses a rubber (PDMS) stamp in which a pattern is moulded from a master Si wafer that is patterned using optical interference lithography or electron beam lithography. The rubber stamp is used to replicate the patterns in a sol-gel layer spin-coated on the Si wafer. The patterned sol-gel layer is then used as a mask for a RIE process that results in the formation of Si nanocylinders in the Si wafer. For this work, master template containing a 4×4 mm 2 array of 250 nm wide, 150 nm high Si NPs with array pitch of 450 nm was fabricated on a 4-inch Si(100) wafer using electron beam lithography and etching. The pattern in the sol-gel was transferred to the Si wafer with two-step RIE: a N 2 and CF 4 gas mixture was used to etch through the sol-gel layer, and N 2 and Cl 2 gases were used to etch the Si wafer. The sol-gel etch mask was removed with diluted HF after which the samples were coated with Si 3 N 4 layers of different thicknesses using low-pressure chemical vapour deposition at 850 ° C. The 4-inch wafer shown in the photograph of Figure 3 was fabricated with a similar process, where the master pillar pattern was made using optical interference lithography with a 266-nm wavelength laser. Optical measurements The total reflectivity spectra in Figure 2c,d were measured in a Labsphere 4-inch integrating sphere, using a supercontinuum broadband light source (Fianium SC450-A, spectral range 0.45–2 μm). The beam spot on the sample was 1 mm in diameter. Light from the integrating spheres was collected with a multimode optical fibre and sent to a spectrometer, comprising a spectrograph (Acton, SpectraPro 300i) and a Si CCD array (Princeton Instruments). The data were confirmed by measurements in a PerkinElmer Lambda950 spectrophotometer, using a tungsten-halogen lamp and deuterium lamp as sources, a PM R6872 detector for the ultraviolet-visible spectral range and a Peltier-cooled PbS detector for near-infrared range. Specular reflectivity for varying AOI ( Fig. 4 and Supplementary Fig. S5 ) was measured in a double-rotation stage (Huber), where the sample was mounted in the inner stage and a power metre (Thorlabs, PM300) on the outer one. For the measurements at the 632 nm wavelength, a Helium-Neon laser source and a Thorlabs LPVIS 100 broadband linear polarizer were used (incident power on the sample: 4 mW); an argon-krypton laser source and a ColorPol VIS500 linear polarizer (10 mW on the sample) were used for the 514 nm wavelength; a diode laser source and a Thorlabs LPUV 050 polarizer (3 mW on the sample) for the 405 nm wavelength. In all cases, the beam spot size on the sample was 1 mm in diameter. How to cite this article: Spinelli, P. et al . Broadband omnidirectional antireflection coating based on subwavelength surface Mie resonators. Nat. Commun. 3:692 doi: 10.1038/ncomms1691 (2012).